Ablation of the p16INK4atumour suppressor reverses ageing phenotypes ofklothomice The p16 INK4a tumour suppressor has an established role in the implementation of cellular senescence in stem/progenitor cells, which is thought to contribute to organismal ageing. However, since p16 INK4a knockout mice die prematurely from cancer, whether p16 INK4a reduces longevity remains unclear. Here we show that, in mutant mice homozygous for a hypomorphic allele of the α-klotho ageing-suppressor gene ( kl kl/kl ), accelerated ageing phenotypes are rescued by p16 INK4a ablation. Surprisingly, this is due to the restoration of α-klotho expression in kl kl/kl mice and does not occur when p16 INK4a is ablated in α-klotho knockout mice ( kl −/− ), suggesting that p16 INK4a is an upstream regulator of α-klotho expression. Indeed, p16 INK4a represses α-klotho promoter activity by blocking the functions of E2Fs. These results, together with the observation that the expression levels of p16 INK4a are inversely correlated with those of α-klotho throughout ageing, indicate that p16 INK4a plays a previously unrecognized role in downregulating α-klotho expression during ageing. Tissue repair and regeneration are essential for longevity in complex animals, and often depend on the proliferative activity of stem or progenitor cells [1] . In many tissues, the proliferative activity of such cells declines with age, contributing to many ageing-associated pathologies [2] , [3] , [4] . In mammals, the p16 INK4a tumour-suppressor gene elicits irreversible cell-cycle arrest known as cellular senescence [5] , [6] , [7] , [8] , [9] , [10] , and its expression increases with age in many tissues [11] , [12] , [13] , along with the accumulation of dysfunctional senescent stem/progenitor cells [14] , [15] , [16] . However, recent studies using middle-aged mice lacking p16 INK4a ( p16 −/− mice) revealed that the ageing-associated induction of p16 INK4a expression reduces the proliferative and regenerative capacities of certain stem/progenitor cells during the ageing process [14] , [15] , [16] . These findings have led to speculation that the induction of p16 INK4a expression and the consequent cellular senescence are causally implicated in ageing-associated declines in stem/progenitor cell functions, thereby reducing longevity. However, since p16 −/− mice die of cancer long before they reach the age at which most normal mice start to die [17] , it remains unclear whether p16 INK4a truly limits longevity in mammals. One approach to circumvent this problem would be the use of short-lived mouse strains with accelerated-ageing phenotypes. However, attempts towards extending the maximum lifespan of accelerated-ageing mouse strains by p16 INK4a ablation have so far been unsuccessful [18] , [19] , raising the question of whether p16 INK4a truly limits longevity in mammals. Mutant mice homozygous for a severely downregulated hypomorphic allele of the α-klotho gene (referred to as kl kl/kl or klotho mice) manifest multiple age-related disorders that are also observed in humans, including infertility, growth retardation, osteoporosis, pulmonary emphysema, skin atrophy, ectopic calcification and shortened lifespan [20] . Furthermore, the levels of α-klotho expression decline with age in both humans and mice [21] , and overexpression of α-klotho extends the maximum lifespan in mice [22] , suggesting that α-klotho acts as an ageing-suppressor gene in mammals [23] . The α-klotho gene encodes a single-pass transmembrane protein that is predominantly expressed in the kidney [20] , and to a lesser extent in the brain [24] . Two forms of the α -klotho protein exist: a membrane-bound form and a secreted form [25] , and each has different functions [22] , [24] , [26] , [27] . As increases in senescent progenitor cells and decreases in stem cell numbers were observed in several tissues in kl kl/kl mice [28] , [29] , we wondered whether p16 INK4a contributes to the accelerated-ageing phenotypes in kl kl/kl mice, by eliciting cellular senescence in certain stem/progenitor cells. In the present study, we explore the roles of p16 INK4a in accelerated-ageing phenotypes of klotho mice. We show that ablation of the p16 INK4a gene reverses various ageing phenotypes, including maximum lifespan, of kl kl/kl mice. Surprisingly, however, this is due to the restoration of α-klotho expression in kl kl/kl mice and does not occur when p16 INK4a is ablated in knockout mice lacking α-klotho ( kl −/− ), indicating that p16 INK4a is an upstream regulator of α-klotho expression. Thus, although p16 INK4a has an established role in the implementation of cellular senescence in stem/progenitor cells [5] , [6] , [7] , [8] , [9] , [10] , which are likely to reduce longevity [13] , our results reveal that p16 INK4a has an additional function in promoting ageing phenotypes by downregulating α-klotho expression in mice. Our findings advance our understanding of the molecular mechanisms underlying the development and progression of ageing in mammals. Ablation of p16 INK4a reverses ageing phenotypes of klotho mice To investigate whether p16 INK4a contributes to the accelerated-ageing phenotypes in kl kl/kl mice, we first generated kl kl/kl mice lacking p16 INK4a ( kl kl/kl p16 −/− mice) by cross-breeding heterozygous klotho ( kl kl/+ ) mice with heterozygous p16 INK4a knockout ( p16 +/− ) mice, and tested whether the accelerated-ageing phenotypes of kl kl/kl mice can be reversed by p16 INK4a ablation. Various accelerated-ageing phenotypes of kl kl/kl mice, such as growth retardation, osteoporosis, pulmonary emphysema and severe atrophy of the intestinal wall and skin, were remarkably mitigated in the kl kl/kl p16 −/− mice as compared with those in the kl kl/kl p16 +/+ (referred to as kl kl/kl ) or kl kl/kl p16 +/− littermates with the same genetic background (98.375% C57BL/6J, 1.625% C3H/J) ( Figs 1 and 2 , and data not shown). Moreover, the maximum lifespan of the kl kl/kl p16 −/− mice was significantly extended as compared with those of the kl kl/kl or kl kl/kl p16 +/− littermates, irrespective of gender ( Fig. 1b , and data not shown). These results indicated that the accelerated-ageing phenotypes of the kl kl/kl mice depend strongly on the p16 INK4a status. The simplest explanation for these results would be that the α -klotho deficiency caused the ageing phenotypes by elevating p16 INK4a expression, and thus p16 INK4a ablation would mitigate the ageing phenotypes in kl kl/kl mice. 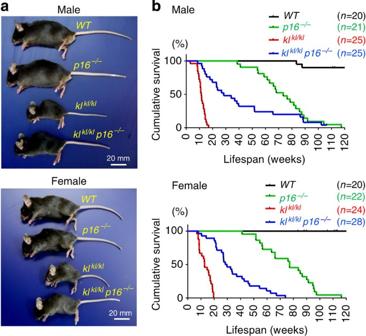Figure 1: Extension of maximum lifespan ofklkl/klmice byp16INK4aablation. (a) Representative photographs of 11-week-old mice of each genotype (n=3). (b) Kaplan–Meier plot showing survival ofWT(male,n=20; female,n=20), p16−/−(male,n=21; female,n=22), klkl/kl(male,n=25; female,n=24) andp16−/−klkl/kl(male,n=25; female,n=28). Figure 1: Extension of maximum lifespan of kl kl/kl mice by p16 INK4a ablation. ( a ) Representative photographs of 11-week-old mice of each genotype ( n =3). ( b ) Kaplan–Meier plot showing survival of WT (male, n =20; female, n =20) , p16 −/− (male, n =21; female, n =22) , kl kl/kl (male, n =25; female, n =24) and p16 −/− kl kl/kl (male, n =25; female, n =28). 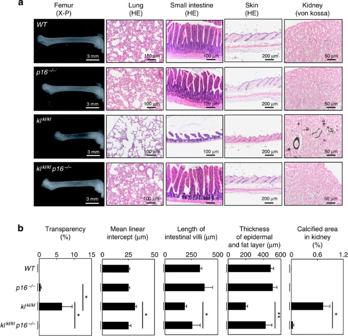Figure 2: Reversing the ageing phenotypes ofklkl/klmice byp16INK4aablation. (a) Histological analysis of 11-week-old femaleWT, p16−/−, klkl/kland p16−/−klkl/klmice. Representative images of bone radiographs of femurs (X-P), HE of tissues indicated top and von Kossa staining (von Kossa) of the kidney for detecting ectopic calcification were shown. (b) The histograms indicate the quantitative analysis of X-ray transparency of femur (WT(n=3), p16−/−(n=3), klkl/kl(n=6) andp16−/−klkl/kl(n=3)), the mean linear intercept (Lm) in lung tissue (WT(n=9), p16−/−(n=9), klkl/kl(n=7) andp16−/−klkl/kl(n=9)), intestinal villi length (WT(n=14), p16−/−(n=7), klkl/kl(n=11) andp16−/−klkl/kl(n=3)), epidermal and subcutaneous fat layer thickness (WT(n=6), p16−/−(n=6), klkl/kl(n=8) andp16−/−klkl/kl(n=3)) and the percentages of calcified areas in kidneys (WT(n=3), p16−/−(n=3), klkl/kl(n=3) andp16−/−klkl/kl(n=3)). For graphs of X-ray transparency of femur and Lm in lung tissues, data were analysed by Mann–WhitneyU-test and are displayed as mean±s.e.m. For graphs of intestinal villi length, epidermal and subcutaneous fat layer thickness and the percentages of calcified areas in kidneys, data were analysed by Student’st-test and are displayed as mean±s.e.m. For all graphs:*P<0.05,**P<0.01. Full size image Figure 2: Reversing the ageing phenotypes of kl kl/kl mice by p16 INK4a ablation. ( a ) Histological analysis of 11-week-old female WT, p16 −/− , kl kl/kl and p16 −/− kl kl/kl mice. Representative images of bone radiographs of femurs (X-P), HE of tissues indicated top and von Kossa staining (von Kossa) of the kidney for detecting ectopic calcification were shown. ( b ) The histograms indicate the quantitative analysis of X-ray transparency of femur ( WT ( n =3) , p16 −/− ( n =3) , kl kl/kl ( n =6) and p16 −/− kl kl/kl ( n =3)), the mean linear intercept (Lm) in lung tissue ( WT ( n =9) , p16 −/− ( n =9) , kl kl/kl ( n =7) and p16 −/− kl kl/kl ( n =9)), intestinal villi length ( WT ( n =14) , p16 −/− ( n =7) , kl kl/kl ( n =11) and p16 −/− kl kl/kl ( n =3)), epidermal and subcutaneous fat layer thickness ( WT ( n =6) , p16 −/− ( n =6) , kl kl/kl ( n =8) and p16 −/− kl kl/kl ( n =3)) and the percentages of calcified areas in kidneys ( WT ( n =3) , p16 −/− ( n =3) , kl kl/kl ( n =3) and p16 −/− kl kl/kl ( n =3)). For graphs of X-ray transparency of femur and Lm in lung tissues, data were analysed by Mann–Whitney U -test and are displayed as mean±s.e.m. For graphs of intestinal villi length, epidermal and subcutaneous fat layer thickness and the percentages of calcified areas in kidneys, data were analysed by Student’s t -test and are displayed as mean±s.e.m. For all graphs: *P <0.05, **P <0.01. Full size image To test this hypothesis, we took advantage of using the p16-luc mice [12] , in which the levels of p16 INK4a expression can be monitored throughout the body using a bioluminescence imaging (BLI) technique. The p16-luc mice were crossed into the klotho genetic background and were subjected to BLI. Unexpectedly, however, we were unable to detect any substantial increase of p16 INK4a expression throughout the body in kl kl/kl mice as judged by BLI ( Fig. 3 ). Because α-klotho is predominantly expressed in the kidney [20] , [24] (see also Supplementary Fig. 1 ), we further examined the p16 INK4a expression in the kidney using quantitative reverse transcription–PCR (qRT–PCR) analysis. Again, however, there was a slight but insubstantial increase of p16 INK4a expression in the kidneys of kl kl/kl mice, as compared with p16 INK4a expression in those of wild-type (wt) mice ( Supplementary Fig. 2 ). These results raise a question of how the p16 INK4a ablation reversed the accelerated-ageing phenotypes of kl kl/kl mice. 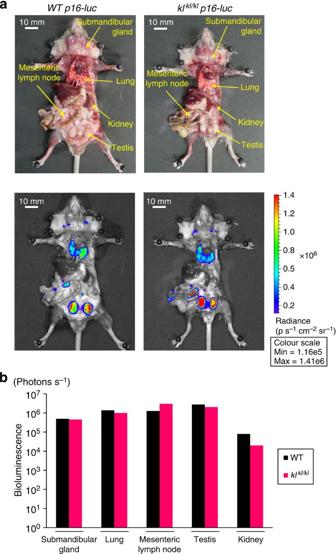Figure 3: Bioluminescencein vivoimaging ofp16INK4aexpression inklkl/klmice. (a) Littermates of 8-week-old malep16-lucmice (WT p16-luc) andp16-lucmice homozygous for a severely downregulated hypomorphic allele of theα-klotho(klkl/klp16-luc) were subjected toin vivobioluminescence imaging after being incised through the throat and the anus under anaesthesia. Representative images of three independent experiments are shown (n=3 experiments). The colour bar indicates photons with minimum and maximum threshold values. (b) Bioluminescence intensity emitted from the organs was graphed (log 10 scale). Figure 3: Bioluminescence in vivo imaging of p16 INK4a expression in kl kl/kl mice. ( a ) Littermates of 8-week-old male p16-luc mice ( WT p16-luc ) and p16-luc mice homozygous for a severely downregulated hypomorphic allele of the α-klotho ( kl kl/kl p16-luc ) were subjected to in vivo bioluminescence imaging after being incised through the throat and the anus under anaesthesia. Representative images of three independent experiments are shown ( n =3 experiments). The colour bar indicates photons with minimum and maximum threshold values. ( b ) Bioluminescence intensity emitted from the organs was graphed (log 10 scale). Full size image p16 INK4a ablation restores α-klotho expression in kl kl/kl mice To explain the effects of the p16 INK4a ablation on the accelerated-ageing phenotypes of kl kl/kl mice, we next took a closer look at the biochemical characteristics of kl kl/kl mice. In kl kl/kl mice, the level of 1α-hydroxylase gene expression is reportedly increased in the kidneys, resulting in an elevated serum level of 1,25-dihydroxyvitamin D, the active metabolite of vitamin D that regulates calcium and phosphate homeostasis [30] . Since these changes are known to be associated with the accelerated-ageing phenotypes in kl kl/kl mice [31] , we examined the levels of these biochemical hallmarks in kl kl/kl mice. Notably, the levels of these hallmarks were substantially reduced in kl kl/kl p16 −/− mice, as compared with those in kl kl/kl mice ( Fig. 4a,b ). Moreover, the aberrant activation of calpain-1 and the ectopic calcification in kidneys, signs of the abnormal calcium homeostasis observed in kl kl/kl mice [20] , [27] , [32] , were absent in kl kl/kl p16 −/− mice ( Figs 2 and 4c ), implying that the α-klotho function might be somewhat restored in the kl kl/kl p16 −/− mice. Since the kl kl/kl mice are not a complete null, but have a severe hypomorphic mutation for α-klotho expression, the entire α-klotho -coding sequence is intact in kl kl/kl mice [20] . Thus, we next wondered whether p16 INK4a ablation could restore the levels of α-klotho expression in kl kl/kl mice. Indeed, the levels of both α-klotho mRNA and protein were substantially increased in the kidneys of kl kl/kl p16 −/− mice, as compared with those in kl kl/kl mice, albeit to lesser extents as compared with those in wt mice ( Fig. 4a,c ). Notably, α-klotho expression was observed only in the renal distal convoluted tubules in kl kl/kl p16 −/− mice ( Fig. 5a ), which are the major sources of α-klotho expression in wt mice [20] . Thus, it appears that p16 INK4a ablation restores the normal α-klotho expression pattern in kl kl/kl mice. Importantly, in stark contrast to the kl kl/kl mice, the p16 INK4a ablation failed to reverse the accelerated-ageing phenotype in mice lacking the α - klotho gene ( α - klotho knockout mice ( kl −/− ; ref. 30 ; Supplementary Fig. 3 ). These results indicate that p16 INK4a ablation mitigates the accelerated-ageing phenotypes of kl kl/kl mice, by restoring α - klotho expression. 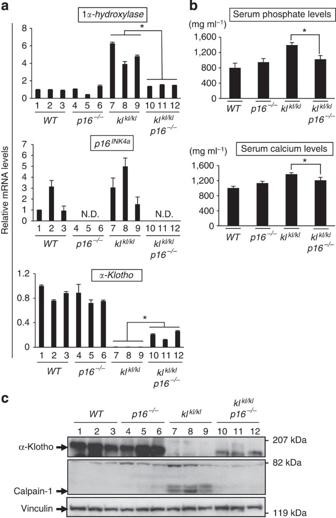Figure 4: Recovery ofα-klothoexpression in the kidney byp16INK4aablation. (a) The relative levels of indicated mRNA in kidneys of 2- to 6-month-old male mice of each genotype were examined using RT–qPCR. Representative results of three individual male mice were shown. N.D. represents ‘not detected’. (b) Serum phosphate and serum calcium levels of 2- to 6-month-old male mice of each genotype were shown. Representative results of three individual mice were shown. (c) Kidneys of each genotype were subjected to western blot analysis using antibodies shown left. Calpain-1 represents the levels of activated form of Calpain-1. Vinculin was used as a loading control. Representative results of three individual male mice were shown. For all graphs, the experiments were performed in triplicate, and representative results from three independent experiments are shown. Data were analysed by Welch’st-test and are displayed as mean±s.d.*P<0.05. Figure 4: Recovery of α-klotho expression in the kidney by p16 INK4a ablation. ( a ) The relative levels of indicated mRNA in kidneys of 2- to 6-month-old male mice of each genotype were examined using RT–qPCR. Representative results of three individual male mice were shown. N.D. represents ‘not detected’. ( b ) Serum phosphate and serum calcium levels of 2- to 6-month-old male mice of each genotype were shown. Representative results of three individual mice were shown. ( c ) Kidneys of each genotype were subjected to western blot analysis using antibodies shown left. Calpain-1 represents the levels of activated form of Calpain-1. Vinculin was used as a loading control. Representative results of three individual male mice were shown. For all graphs, the experiments were performed in triplicate, and representative results from three independent experiments are shown. Data were analysed by Welch’s t -test and are displayed as mean±s.d. *P <0.05. 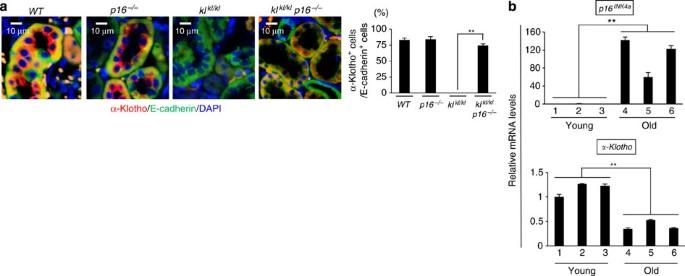Figure 5: Inverse correlation betweenα-klothoandp16INK4aexpression. (a) Immunohistochemical analysis ofα-klotho (red), E-cadherin (green) and 4,6-diamidino-2-phenylindole (blue) in 11-week-old male mouse kidney sections of each genotype. Representative results of three individual male mice were shown. The histograms indicate the percentages of E-cadherin-expressing cells that were positive forα-klotho expression. At least 100 cells were scored per group. (b) The relative levels of indicated mRNA in kidneys of young (10- to 20-week-old) or old (120- to 140-week-old)Wtmale mice were examined using RT–qPCR. Representative results of three individual male mice were shown. For all graphs, the experiments were performed in triplicate, and representative results from three independent experiments are shown. Data were analysed by Welch’st-test and are displayed as mean±s.d.*P<0.05,**P<0.01. Full size image Figure 5: Inverse correlation between α-klotho and p16 INK4a expression. ( a ) Immunohistochemical analysis of α -klotho (red), E-cadherin (green) and 4,6-diamidino-2-phenylindole (blue) in 11-week-old male mouse kidney sections of each genotype. Representative results of three individual male mice were shown. The histograms indicate the percentages of E-cadherin-expressing cells that were positive for α -klotho expression. At least 100 cells were scored per group. ( b ) The relative levels of indicated mRNA in kidneys of young (10- to 20-week-old) or old (120- to 140-week-old) Wt male mice were examined using RT–qPCR. Representative results of three individual male mice were shown. For all graphs, the experiments were performed in triplicate, and representative results from three independent experiments are shown. Data were analysed by Welch’s t -test and are displayed as mean±s.d. *P <0.05, **P <0.01. Full size image p16 INK4a downregulates α-klotho expression in wt mice The obvious next question is whether p16 INK4a downregulates α-klotho expression in wt mice. Note that there is an inverse correlation between the levels of p16 INK4a expression and α-klotho expression during the ageing process in kidneys ( Fig. 5b ). However, because p16 −/− mice die prematurely from cancer [17] (see also Fig. 1b ), we cannot examine whether p16 INK4a ablation ameliorates the ageing-associated decline of α-klotho expression in mice harbouring wt α-klotho . To circumvent this problem, we employed the mouse model of chemically induced kidney injury. It was previously reported that patients with chronic renal failure develop multiple age-related disorders resembling those of kl kl/kl mice, with a marked reduction of α-klotho expression in kidneys [33] , [34] . Moreover, treatment with cisplatin, a chemotherapeutic agent that causes severe adverse actions with nephrotoxicity, is known to provoke a significant reduction of α - klotho expression in kidneys, accompanied by the accumulation of DNA damage [35] . Since persistent DNA damage induces p16 INK4a expression in many different cell types [12] , we analysed the effect of p16 INK4a expression on the levels of α - klotho expression in the cisplatin-induced kidney injury model. Indeed, the cisplatin treatment resulted in a marked reduction of α - klotho expression in the renal distal convoluted tubules of wt mice, coinciding with the accumulation of γH2AX foci, a sign of the DNA damage response, and the induction of p16 INK4a expression ( Supplementary Fig. 4 ). Notably, however, the cisplatin-induced reduction of α - klotho expression was substantially attenuated in the p16 −/− mice ( Supplementary Fig. 4 ), although this level of α - klotho restoration was insufficient to block the cisplatin-induced nephrotoxicity in this experimental condition ( Supplementary Fig. 5 ), indicating that p16 INK4a has the potential to downregulate α-klotho expression in wt mice as well. p16 INK4a downregulates the α - klotho promoter in murine cells To further verify this notion, we next sought evidence that p16 INK4a downregulates α - klotho promoter activity. As α-klotho expression is rather limited in the renal distal convoluted tubules [20] , [24] , we were unable to find any established murine cell lines expressing substantial levels of α-klotho ( Supplementary Fig. 6 ). Therefore, primary m ouse r enal t ubular e pithelial c ell s (mRTECs) were prepared from the kidneys of wt mice, and were used for a promoter–reporter analysis. The luciferase activity of a reporter plasmid containing the region 1,035 nucleotides upstream of the mouse α-klotho translation start site was reduced by the ectopic expression of p16 INK4a in a dose-dependent manner in early-passage primary mRTECs ( Fig. 6a ), indicating that p16 INK4a indeed downregulates α-klotho expression at the promoter level. Although the α-klotho promoter sequences are not well conserved between human and mouse, both include potential binding sites for E2F transcription factors, which are critical downstream mediators of the p16 INK4a –retinoblastoma tumour suppressor pathway [6] , at the same position from the α-klotho translation start sites ( Figs 6a and 7b ). Notably, newborn mice lacking both E2F1 and E2F3a, a subset of the activator E2Fs (referred to as E2F1 −/− E2F3a −/− mice), reportedly exhibited normal weight and appearance; however, by their third week of life the proliferative index of most tissues was significantly reduced, and 90% of the mice became severely runted and died within 2 months [36] . Furthermore, white adipose tissues were absent and lung alveolar branching was severely reduced in E2F1 −/− E2F3a −/− mice [36] . Since these phenotypes are reminiscent of the kl kl/kl phenotypes [20] , we analysed whether E2F1 and/or E2F3 activate the α-klotho promoter activity. Indeed, the ectopic expression of either E2F1 or E2F3 increased the activity of the α-klotho promoter in cultured primary mRTECs ( Fig. 6b ). However, this was not the case when the E2F-binding element was disrupted by a nucleotide substitution in the reporter plasmid ( Fig. 6b , -674 E2F-Mut). Moreover, increasing amounts of E2F3 blocked the trans -repressing activity of co-transfected p16 INK4a in early-passage primary mRTECs ( Supplementary Fig. 7 ). Note that endogenous E2F1 and E2F3 were found to bind to the α-klotho promoter, as judged by a chromatin immunoprecipitation (ChIP) analysis using cultured primary mRTECs or kidney tissues prepared from wt mice ( Fig. 6c ). These results, in conjunction with the observation that the levels of endogenous α-klotho mRNA and protein expression were substantially reduced in the kidneys of E2F1 −/− E2F3a −/− mice ( Fig. 6d ), strongly suggest that p16 INK4a downregulates α-klotho expression, at least partly by blocking the function of activator E2Fs in wt mice. 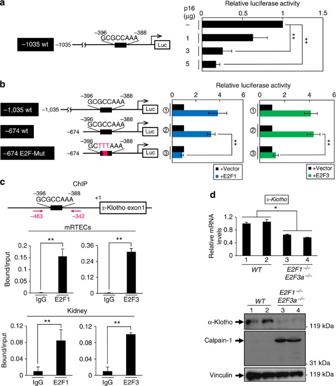Figure 6: p16INK4adownregulatesα-klothogene promoter activityviaE2F. (a,b) Schematic representation of the reporter construct of mouseα-klothogene promoter used in the analysis (left panel). The E2F-binding element is shown as a black rectangle with the sequence and firefly luciferase is shown as Luc. The reporter construct was co-transfected into mRTECs along with LacZ or Renilla plasmid. Where indicated, cells were also co-transfected with an increasing amount of p16INK4aexpression plasmid (a) or with 2 μg of expression plasmid encoding E2F1 or E2F3 (b). (c) Early-passage mRTECs and kidney tissues were prepared from 6- to 10-week-old male mice and were subjected to ChIP analysis using antibodies shown at bottom and PCR primers shown at the top (red arrows). (d) The relative levels ofα-klothomRNA and protein expression in kidneys of each genotype were examined using RT–qPCR (upper panel) or western blot analysis (lower panel). Representative results of two individual 2.7-week-old male mice were shown. For all graphs, the experiments were performed in triplicate, and representative results from three independent experiments are shown. Data were analysed by Welch'st-test and are displayed as mean±s.d.*P<0.05,**P<0.01. Figure 6: p16 INK4a downregulates α-klotho gene promoter activity via E2F. ( a , b ) Schematic representation of the reporter construct of mouse α-klotho gene promoter used in the analysis (left panel). The E2F-binding element is shown as a black rectangle with the sequence and firefly luciferase is shown as Luc. The reporter construct was co-transfected into mRTECs along with LacZ or Renilla plasmid. Where indicated, cells were also co-transfected with an increasing amount of p16 INK4a expression plasmid ( a ) or with 2 μg of expression plasmid encoding E2F1 or E2F3 ( b ). ( c ) Early-passage mRTECs and kidney tissues were prepared from 6- to 10-week-old male mice and were subjected to ChIP analysis using antibodies shown at bottom and PCR primers shown at the top (red arrows). ( d ) The relative levels of α-klotho mRNA and protein expression in kidneys of each genotype were examined using RT–qPCR (upper panel) or western blot analysis (lower panel). Representative results of two individual 2.7-week-old male mice were shown. For all graphs, the experiments were performed in triplicate, and representative results from three independent experiments are shown. Data were analysed by Welch's t -test and are displayed as mean±s.d. *P <0.05, **P <0.01. 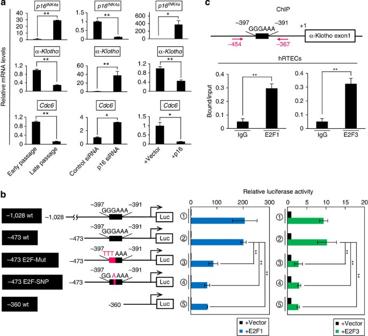Figure 7: p16INK4adownregulatesα-klothoexpression in humans. (a) The relative levels of indicated mRNA in hRTECs were examined using RT–qPCR. RNAs were prepared from early-passaged or late-passaged hRTECs (left panels), early-passaged hRTECs transfected with siRNA against p16INK4aor control (middle panels), or early-passaged hRTECs transfected with or without p16INK4aexpression vector (right panels). (b) Schematic representation of the reporter construct of the humanα-klothogene promoter used in the analysis (left panel). The E2F-binding element is shown as a black rectangle with the sequence and firefly luciferase is shown as Luc. The reporter construct was co-transfected into hRTECs along with Renilla plasmid. Where indicated, cells were also co-transfected with 1.5 μg of expression plasmid encoding E2F1 or E2F3. (c) Early-passage cultured hRTECs were subjected to ChIP analysis using antibodies shown at bottom and PCR primers shown at the top (red arrows). For all graphs, the experiments were performed in triplicate, and representative results from three independent experiments are shown. Data were analysed by Welch'st-test and are displayed as mean±s.d.*P<0.05,**P<0.01. Full size image Figure 7: p16 INK4a downregulates α-klotho expression in humans. ( a ) The relative levels of indicated mRNA in hRTECs were examined using RT–qPCR. RNAs were prepared from early-passaged or late-passaged hRTECs (left panels), early-passaged hRTECs transfected with siRNA against p16 INK4a or control (middle panels), or early-passaged hRTECs transfected with or without p16 INK4a expression vector (right panels). ( b ) Schematic representation of the reporter construct of the human α-klotho gene promoter used in the analysis (left panel). The E2F-binding element is shown as a black rectangle with the sequence and firefly luciferase is shown as Luc. The reporter construct was co-transfected into hRTECs along with Renilla plasmid. Where indicated, cells were also co-transfected with 1.5 μg of expression plasmid encoding E2F1 or E2F3. ( c ) Early-passage cultured hRTECs were subjected to ChIP analysis using antibodies shown at bottom and PCR primers shown at the top (red arrows). For all graphs, the experiments were performed in triplicate, and representative results from three independent experiments are shown. Data were analysed by Welch's t -test and are displayed as mean±s.d. *P <0.05, **P <0.01. Full size image p16 INK4a downregulates α - klotho expression in human cells Finally, to further support our murine data and to extend the analysis to human physiology, we tested whether p16 INK4a downregulates α - klotho mRNA expression in human cells. Similar to murine cells, primary human RTECs (hRTECs), but not other human cell lines, express substantial levels of α - klotho ( Supplementary Fig. 8 ). We thus used primary hRTECs in the following experiments. We found that the levels of α - klotho mRNA expression declined when cultured primary hRTECs were rendered senescent by serial passage, accompanied by the induction of p16 INK4a mRNA expression ( Fig. 7a , left). However, the short interfering RNA (siRNA)-mediated depletion of p16 INK4a substantially increased the levels of α - klotho mRNA expression in late-passage hRTECs, coinciding with the increased expression of cdc6, an established E2F target gene ( Fig. 7a , middle). Conversely, the ectopic expression of p16 INK4a reduced the levels of α - klotho mRNA expression in early-passage hRTECs ( Fig. 7a , right). Together, these results suggest that p16 INK4a downregulates α-klotho expression, by blocking the function of the activator E2Fs in human cells, as well as in mouse cells. Indeed, the ectopic expression of either E2F1 or E2F3 substantially increased the transcriptional activity of the human α-klotho promoter in cultured hRTECs ( Fig. 7b , −1,028 wt and −473 wt). These effects were blunted when the putative E2F-binding site within the human α-klotho promoter was mutated or deleted in the reporter plasmid ( Fig. 7b , -473 E2F-Mut and-360 wt). Furthermore, the ChIP analysis revealed that endogenous E2F1 and E2F3 bind to the human α-klotho promoter in cultured hRTECs ( Fig. 7c ). Interestingly, the G to A single-nucleotide polymorphism (SNP), in the putative E2F-binding site of the human α-klotho promoter, reportedly impaired the DNA–protein interaction and is associated with the reduction of bone mineral density (BMD) in aged postmenopausal women [37] . Indeed, the G to A substitution in the E2F-binding site of the reporter plasmid greatly reduced the response to E2F overexpression ( Fig. 7b ,-473 E2F-SNP). These results, in conjunction with previous observations that there is the potential inverse correlation between the levels of renal p16 INK4a expression and α -klotho expression in elderly people [21] , [38] , [39] , [40] , suggest that p16 INK4a is likely to have the potential to downregulate α-klotho expression by blocking the transcriptional activity of E2Fs in human kidneys. The ageing process is multifactorial, with genetic background and environmental stress as two critical components [4] , [41] . The mutation of the α-klotho gene causes multiple premature ageing phenotypes, including a shortened lifespan in mice [20] , and some SNPs in the human α-klotho gene are associated with reduced lifespans [37] , [42] , [43] . Moreover, the levels of plasma α -klotho decrease with increasing age and are associated with longevity in humans [21] , [40] , indicating that the α-klotho gene is an important antiageing gene in both mouse and human. However, it remained unclear how the α-klotho gene could be linked to environmental stress. Here we show that the p16 INK4a tumour-suppressor gene, a stress sensor known to induce cellular senescence [5] , [6] , [7] , [8] , [9] , [10] , [11] , [12] , downregulates α-klotho gene expression in both mouse and human renal tubular epithelial cells. Ablation of the p16 INK4a gene mitigates various accelerated-ageing phenotypes of kl kl/kl mice, including shortened maximum lifespan, by partially restoring α - klotho expression ( Figs 1 , 2 and 4 ). Furthermore, cell culture studies reveal that p16 INK4a represses α - klotho gene expression at the promoter level by blocking the function of activator E2F, most likely through activation of retinoblastoma protein in mouse and human cells ( Figs 6 , 7 , 8 ). These results, together with previous epidemiological studies [38] , [39] , suggest that this previously unrecognized function of p16 INK4a is likely to play a role in humans as well as in mice. 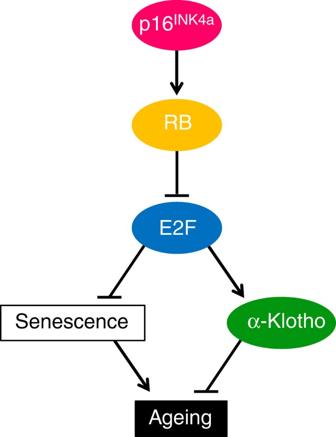Figure 8: Dual roles for the p16INK4aRB pathway in organismal ageing. The p16INK4ahas an established role in provoking cellular senescence, which is likely to cause stem cell ageing and thereby contributing to organismal ageing. Here we show that, in addition, p16INK4aalso contributes to organismal ageing through blocking the expression of ageing suppressor,α-klotho. Figure 8: Dual roles for the p16 INK4a RB pathway in organismal ageing. The p16 INK4a has an established role in provoking cellular senescence, which is likely to cause stem cell ageing and thereby contributing to organismal ageing. Here we show that, in addition, p16 INK4a also contributes to organismal ageing through blocking the expression of ageing suppressor, α -klotho. Full size image However, p16 INK4a has an established role in the implementation of cellular senescence in stem/progenitor cells [5] , [6] , [7] , [8] , [9] , [10] , thereby causing dysfunctional tissue regeneration and repair [13] , which are likely to reduce longevity. Indeed, a series of studies using middle-aged p16 −/− mice revealed that the ageing-associated induction of p16 INK4a expression reduces the proliferative and regenerative capacities of certain progenitor cells during the ageing process [14] , [15] , [16] , further illustrating the importance of the p16 INK4a -cellular senescence pathway in the development of ageing phenotypes [44] . Nevertheless, our present study revealed that p16 INK4a plays another role in promoting ageing phenotypes, through the downregulation of the expression of the α -klotho ageing suppressor (see model in Fig. 8 ). This previously unrecognized pathway, linking p16 INK4a to α-klotho expression, enhances our understanding of the molecular mechanisms underlying the development and progression of ageing phenotypes in mammals and opens up new possibilities for their control. Mice All efforts were made to minimize animal suffering and to reduce the number of animals used. Wt mice (C57BL/6J), klotho ( kl kl/kl ) mice [20] (mixed C57BL/6J and C3H/J genetic background; 50% C57BL/6J, 50% C3H/J) and α - klotho knockout ( kl −/− ) mice (C57BL/6J) were purchased from CLEA Inc., Japan. Kl kl/kl mice were backcrossed with C57BL/6J mice for five generations and used in this study. Kl kl/kl p16-luc mice were generated by crossing kl kl/kl mice with p16-luc mice [12] . E2F1 −/− E2F3 −/− mice [36] were provided by Dr Gastabo Leone. p16 −/− mice [45] were provided by Dr Norman E. Sharpless. These mice were maintained under specific pathogen-free conditions, on a 12-h light–dark cycle and fed normal diet (CE-2 from CLEA Inc., composed of 12 kcal% fat, 29 kcal% protein and 59 kcal% carbohydrates). All animal experiments were cared for by protocols approved by the Committee for the Use and Care of Experimental Animals of the Japanese Foundation for Cancer Research. Bone radiography BMD was analysed using X-ray radiography. Femur and tibia were resected from 11-week female mice, and placed on wrapped films (FUJIFILM INDUSTRIAL X-RAY FILM ENVELOPAK IX FR; FUJIFILM Corporation, Japan), and exposed to X-irradiation at 20 kVp, 9 mA for 15 s using a SOFTEX CMB-2 (SOFTEX CO., LTD., Japan). Films were developed using a Fuji Medical Films Processor SEPROS SV (FUJIFILM Corporation) and inspected for BMD. Bioluminescence imaging For the detection of luciferase expression, mice were anaesthetized, injected intraperitoneally with D-luciferin sodium salt (75 mg kg −g ) 5 min before beginning photon recording. Mice were placed in the light-tight chamber and a grey-scale image of the mice was first recorded with dimmed light followed by acquisition of luminescence image using a cooled CCD (charged-coupled device) camera (PIXIS 1024B; Princeton Instruments) [12] , [46] . The signal-to-noise ratio was increased by 2 × 2 binning and 5-min exposure. For colocalization of the luminescent photon emission on the animal body, grey scale and pseudo-colour images were merged by using IMAGE-PRO PLUS (Media Cybernetics). Histology and immunofluorescence analysis Samples were fixed in 10% formalin for a 24 h or longer, progressively dehydrated through gradients of alcohol and embedded in paraffin. Samples were then sectioned on a microtome (5-μm thick), deparaffinized in xylene, rehydrated and then stained with haematoxylin and eosin (HE). For immunofluorescence, the relevant Alexa Fluor 488 goat anti-mouse or 546 goat anti-rabbit antibodies (1:1,000, Molecular probes) were used for detection of primary antibodies. Fluorescence images were observed and photographed using an immunofluorescence microscope (Carl Zeiss). The primary antibodies used for mouse samples were as follows: Klotho (1:100, TransGenic Inc., KO603), E-cadherin (1:100, Cell Signaling no. 3195), γ-H2AX (1:100, Millipore, 05-636). E-cadherin was used as a marker of the renal distal tubes [47] , [48] , [49] . Calcium deposition was visualized with the von Kossa staining. Paraffin-embedded sections were deparaffinized and rehydrated. Fixed sections were incubated with 5% silver nitrate during exposure to light for 60 min, and washed with distilled water. Excess silver was washed out with 5% sodium thiosulfate for 2 min. The sections were then stained with Kernechtrot dye. Epidermal and subcutaneous fat-layer thickness and intestinal villi length were determined using 10–74 random measurements along the length of skin and small intestine from at least three mice per age group and genotype. For skin sections, the skin was cut parallel to the spine and sections were cut perpendicular to the skin surface. For villi sections, intestinal tracts were flushed with PBS and rolled up in a compact circle using longitudinally oriented jejunal sections for analysis; 5-μM sections were used for HE staining, and the Image J software was used for length measurements [50] . The mean linear intercept (Lm) in the lung tissue was calculated using light microscopy and Image J software. An overlay consisting of horizontal and vertical, parallel lines was placed over the photographed image of each region. All intercepts with alveolar septal tissue were counted. The total length of all the lines together divided by the number of intercepts gives the Lm for the region studied. The overall mean of the Lm for each of the three regions studied for each tissue block was used as the Lm for the corresponding tissue block [51] . Reverse transcription and quantitative real-time PCR Total RNA was extracted from mouse tissues using TRIzol reagent (Life Technologies). Reverse transcription and quantitative real-time PCR (RT–qPCR) was performed using the SYBER Premix EX Taq system (TAKARA) and a Prism 7900HT (ABI) [52] , [53] . Amplified signals were confirmed to be single bands with gel electrophoresis and were normalized to the levels of glyceraldehyde 3-phosphate dehydrogenase. The data were analysed using the SDS2.1 software (ABI) [46] . The PCR primer sequences used are shown in the Supplementary Table 1 . Measurement of serum phosphate, calcium and BUN The concentration of serum phosphate, calcium and blood urea nitrogen (BUN) was measured with a phosphate assay kit (Serotec UPi-L; Serotec Co. Ltd., Japan), a calcium assay kit (Metalloassay Ca-CPZIII; AKJ Global Technology, Japan) and a BUN assay kit (Iatoro LQ UN rate (A) II; LSI medience Co. Ltd., Japan), respectively, according to the manufacturers’ instruction. Cell culture For primary mRTECs [47] , kidneys of 6- to 10-week-old male mice were taken and placed in cold PBS containing antibiotics (Penicillin and streptomycin). The medulla of the kidneys were removed and the cortex of the kidney was taken, minced and transferred to 2 ml serum-free DMEM containing 0.1% collagenase (Sigma). Minced kidney cortex tissue was incubated at 37 °C with shaking for 30 min. The tissue suspension was mixed with 10 ml of DMEM containing 10% serum to inactivate collagenase. The remaining tissue mass was removed through the 70-μm strainer, and cells were pelleted using centrifugation. The cell number was counted and seeded on the poly-L-lysin-coated dishes (Corning, USA) for ChIP analysis or for transfection. For normal hRTECs, primary hRTECs were purchased from Lonza (Lonza, Switzerland) and were cultured according to the manufacturer’s instruction. Western blot analysis Tissue lysates were prepared using a homogenizer in lysis buffer (50 mM HEPES (pH 7.5), 150 mM NaCl, 1 mM EDTA, 2.5 mM EGTA, 10% glycerol, 0.1% Tween 20 and 10 mM β-glycerophosphate) containing protease inhibitor cocktail (Nacalai tesque) [54] . The transferred membranes were immunoblotted directly with following antibodies, and the signals were detected using enhanced chemiluminescence system (GE Healthcare). The first antibodies used were as follows: α -Klotho (1:500, TransGenic Inc., KO603), Calpain-1 (μ-Calpain; 1:1,000, Enzo ALX-804-050-R100), α-tubulin (1:1,000, Sigma T9026) and Vinculin (1:1,000, Sigma V9131). Expanded immunoblots are shown in Supplementary Figs 9–11 . ChIP analysis ChIP analysis was performed using the EZ-ChIP kit (Millipore) according to the manufacturer’s instruction. The immunoprecipitation of cross-linked chromatin was conducted with anti-mouse E2F1 (1:1,000, Santa Cruz, sc-193X), anti-mouse E2F3 (1:1,000, Santa Cruz, sc-878X), anti-human E2F1 (1:1,000, Santa Cruz, sc-193X), anti-human E2F3 (1:1,000, Santa Cruz, sc-878X) and rabbit IgG (1:1,000, Cell Signaling Technology, 2729) as a negative control. After immunoprecipitation, DNA was extracted using the QIAquick PCR purification kit (Qiagen) and an aliquot was amplified using qPCR using following primers flanking the putative mouse E2F-binding site position at −388 to −396 bp of mouse α-klotho gene promoter: 5′-TGTTCTCTGAAAGATTCCCC-3′ and 5′-TCCCTTTGCCTTCCTGGGAC-3′, or primers flanking the putative human E2F-binding site position at −391 to −397 bp of human α-klotho gene promoter: 5′-TGGGAGAAAAGTGAGAGCAG-3′ and 5′-TGGGAGAAAAGTGAGAGCAG-3′. In vivo ChIP analysis Sixty milligrams of kidney tissue was chopped into 1- to 2-mm pieces using razor blades and were transferred into a new tube containing 1 ml PBS with proteinase inhibitor cocktail (Nacalai tesque). Crosslinking was performed in 1% of formaldehyde by rotating at room temperature for 15 min. This crosslinking reaction was stopped by adding fresh glycine to a final concentration of 0.125 M by continuous rotation at room temperature for 5 min. Tissue pieces were then washed and suspended in PBS-containing proteinase inhibitor cocktail, and were grinded by Dounce homogenizing seven times. The cell pellet was resuspended into Lysis buffer containing 5 mM PIPES pH8.0, 85 mM KCl, 0.5% NP40 and proteinase inhibitor cocktail, and lysed by Dounce homogenizing four times to aid in nuclei release [52] . After this procedure, ChIP was performed using the EZ-ChIP kit (Millipore). The immunoprecipitation of cross-linked chromatin was conducted with anti-mouse E2F1 (1:1,000, Santa Cruz, sc-193X), anti-mouse E2F3 (1:1,000, Santa Cruz, sc-878X) and rabbit IgG (1:1,000, Cell Signaling Technology, 2729) as a negative control. After immunoprecipitation, DNA was extracted using the QIAquick PCR purification kit (Qiagen), and an aliquot was amplified by qPCR using the following primers flanking the putative mouse E2F-binding site position at −388 to −396 bp of mouse α - klotho gene promoter: 5′-TGTTCTCTGAAAGATTCCCC-3′ and 5′-TCCCTTTGCCTTCCTGGGAC-3′. RNA interference RNA interference (RNAi) was performed using the RNAiMAX transfection reagent (Life Technologies) and siRNA oligos against target genes [53] . The sequences of targeting oligo are as follows. Human p16 5′-GAGGAGGUGCGGGCGCUGCTT-3′ (sense) and 5′-GCAGCGCCCGCACCUCCUCTT-3′ (antisense) Control 5′-AUGAACGUGAAUUGCUCAATT-3′ (sense) and 5′-UUGAGCAAUUCACGUUCAUTT-3′ (antisense). Luciferase–reporter assays The human and mouse α-klotho gene promoter sequence was amplified with PCR using genomic DNA extracted from the mouse tail or BAC clone (RP11-720E2) containing the entire human α-klotho gene as templates. Deletion mutants were prepared with standard PCR procedures. Promoter sequences containing point mutations were generated using the Quick Change Site-directed Mutagenesis kit (Agilent Technologies). The promoter fragments were inserted into PGL3 basic firefly luciferase reporter plasmid (Promega). All inserted DNAs were sequenced and verified. Transfection of reporter plasmids was performed using the X-treamGENE9 DNA transfection reagent (Roche) according to the manufacturer’s instructions. The luciferase assays were performed using the Luciferase assay systems kit (Promega). Cytomegalovirus promoter-renilla luciferase plasmid or SV40 promoter-β-galactosidase plasmid was used as an internal control. Cisplatin ( cis -diamminedichloro-platinum II) treatment Cisplatin was purchased from Wako pure chemical, Japan and dissolved in saline. Mice were intraperitoneally injected with Cisplatin solution (12 mg kg −g ) three times (every other day) for a week and killed. The kidneys were immediately taken from mice and used for analysis. Statistical analysis The significance of differences was analysed by Student’s t -test, Welch's t -test or Mann–Whitney U -test. P values of less than 0.05 were considered to be significant. Statistical analyses were performed using the GraphPad Prism programme Ver. 5.01 ( GraphPad Software Inc.). How to cite this article: Sato, S. et al. Ablation of the p16 INK4a tumour suppressor reverses ageing phenotypes of klotho mice. Nat. Commun. 6:7035 doi: 10.1038/ncomms8035 (2015).